The stress-responsive geneATF3regulates the histone acetyltransferase Tip60 Tat-interactive protein 60 (Tip60) is a MYST histone acetyltransferase that catalyses acetylation of the major DNA damage kinase Ataxia telangiectasia mutated (ATM), thereby triggering cellular signalling required for the maintenance of genomic stability on genotoxic insults. The Tip60 activity is modulated by post-translational modifications that alter its stability and its interactions with substrates. Here we report that activating transcription factor 3 (ATF3), a common stress mediator and a p53 activator, is a regulator of Tip60. ATF3 directly binds Tip60 at a region adjacent to the catalytic domain to promote the protein acetyltransferase activity. Moreover, the ATF3–Tip60 interaction increases the Tip60 stability by promoting USP7-mediated deubiquitination of Tip60. Consequently, knockdown of ATF3 expression leads to decreased Tip60 expression and suppression of ATM signalling as evidenced by accumulated DNA lesions and increased cell sensitivity to irradiation. Our findings thus reveal a previously unknown function of a common stress mediator in regulating Tip60 function. In addition to regulating transcription and controlling cell growth, the MYST histone acetyltransferase Tat-interactive protein 60 (Tip60) acetylates both histones and non-histone proteins, and plays crucial roles in sensing DNA damage, altering chromatin structures and triggering repair signalling that is often mediated by the protein kinase Ataxia telangiectasia mutated (ATM) in response to DNA double-strand breaks [1] . Tip60 achieves these functions by relocating to damage sites, binding to methylated histone H3 (ref. 2 ), and, most importantly, acetylating ATM at lysine 3016 leading to its autophosphorylation, which in turn converts the inactive ATM dimer to an active, monomeric kinase [3] , [4] . ATM then phosphorylates multiple DNA damage response proteins that recruit the DNA repair machinery (for example, H2X), arrest cell cycle progression to allow DNA repair (for example, p53) or induce apoptotic cell death (for example, Chk2 and p53). Tip60 also facilitates DNA-damage repair by recruiting ribonucleotide reductase to increase the deoxynucleoside triphosphate pool [5] , or promoting the exchange of phosphorylated H2AX (γ-H2AX) with unphosphorylated H2AX at repaired sites [6] . Moreover, Tip60 appears to determine the cell fate on genotoxic stress by acetylating the tumour suppressor p53 at lysine 120, thereby selectively promoting pro-apoptotic gene (for example, PUMA) expression [7] , [8] . It is therefore essential for the cell to tightly regulate Tip60 expression and its histone acetyltransferase (HAT) activity in order to maintain genomic integrity and evade from malignant transformation in the face of genotoxic insults. Indeed, partial inactivation of Tip60 in mice (Tip60 +/− ) is sufficient to abrogate oncogene-induced DNA-damage response, thereby accelerating Myc-induced lymphomagenesis [9] . The Tip60 activity is mainly regulated by post-translational modifications. Whereas Tip60 phosphorylation by GSK-3 or c-Abl, or deacetylation by SIRT1, has been shown to alter its HAT activity [10] , [11] , [12] , Tip60 appears to be a relatively unstable protein and is degraded by ubiquitin-dependent proteolysis mediated by the E3 ubiquitin ligase MDM2 and Cullin3 (refs 13 , 14 ). MDM2 directly binds to and adds ubiquitin moieties to Tip60 to promote its degradation [13] . In contrast, Cullin3 requires an adaptor protein, activating transcription factor 2 (ATF2), to degrade Tip60—an effect that can be attenuated by γ-irradiation (IR) [14] . Several viral proteins (for example, HPV E6 and HIV Tat) can also mediate Tip60 degradation through ubiquitination-dependent mechanisms [15] , [16] . On the other hand, the deubiquitinase USP7 was recently shown to bind Tip60 and remove polyubiquitin chains from Tip60, thereby stabilizing the acetyltransferase [17] , [18] . USP7 is one of the best studied deubiquitinases and also contributes to the DNA damage response through regulating the stability of MDM2 or p53 (ref. 19 ). Given the crucial roles of Tip60 in the cellular response to genotoxic stress, it is of great interest to better understand the mechanisms by which the Tip60 activity is regulated. Activating transcription factor 3 (ATF3) belongs to the ATF/CREB transcription factor family that is largely diversified in size, protein sequence and biological function [20] . These proteins only share structural similarity in the basic-region leucine zipper domain, which presumably mediates binding to a consensus DNA sequence (the ATF/CREB cis -element) for transcription regulation. However, it has also been shown that the ATF/CREB proteins possess various biological functions independent of their transcriptional activities. ATF3, for instance, can directly interact with several key cancer-associated proteins (for example, p53, E6, androgen receptor and p63) [21] , [22] , [23] , [24] , and regulate their activities by altering their interactions with DNA or other proteins. Distinct from other ATF/CREB proteins, ATF3 expression is rapidly induced by a wide range of cellular stresses including nutrient deprivation, oxidative stress and DNA damage [25] . Given the fact that the induction of ATF3 expression by DNA damage has been well documented, it is often speculated that this common stress mediator is required for mounting appropriate cellular responses to alleviate potential damages from genotoxic challenges. However, neither the mechanisms by which ATF3 is induced nor the consequences of ATF3 induction has been well elucidated. Whereas ATF3 was shown to transactivate p15 PAF required for eliminating DNA adducts induced by ultraviolet stress [26] , the findings that ATF3 activates p53 by blocking MDM2-mediated ubiquitination and that ATF3 interacts with both p53 and MDM2 (refs 27 , 28 ) argue for the notion that ATF3 likely fine-tunes the p53 activity and thus contributes to the maintenance of genomic integrity. Here we report that ATF3 is a novel Tip60 regulator that promotes not only the HAT activity but the Tip60 stability through binding to Tip60. Consistent with these results, knockdown of ATF3 expression leads to decreased Tip60 expression and impaired ATM activation on IR. These findings thus unveil a novel, pivotal role that ATF3 plays in the regulation of Tip60 activity and subsequent signalling essential for the maintenance of genomic stability on genotoxic stress. ATF3 binds Tip60 under both basal and stressed conditions Given the crucial role of Tip60 in regulating the DNA damage response, we sought to explore whether ATF3 binds Tip60 and alters its activity. Reciprocal co-immunoprecipitation (co-IP) experiments using p53-null H1299 cells showed that ATF3 and Tip60 existed in the same immunocomplex (Fig. 1a,b , lane 3), suggesting that ATF3 might directly bind Tip60. Indeed, whereas the immobilized GST (glutathione S -transferase)–ATF3 protein pulled down in vitro -translated Tip60 ( Fig. 1c , lane 3), GST–Tip60 could also pull down the purified, recombinant ATF3 protein ( Fig. 1d , lane 2). As the commercially available Tip60 antibodies did not work well to precipitate the endogenous Tip60 protein, we determined the interaction between the endogenous Tip60 and ATF3 proteins using an engineered HCT116 cell line (HCT116-3 × FLAG) in which a sequence encoding a 3 × FLAG peptide was added to 3′-end of the native Tip60 gene [18] . The recombinant cells thus express the endogenous Tip60 protein with the 3 × FLAG peptide fused to its C terminus, and accordingly, the endogenous Tip60 can be recognized by a FLAG antibody. Employing these cells, we found that the FLAG antibody could precipitate ATF3 along with the FLAG-tagged Tip60 protein ( Fig. 1e )—a result demonstrating that the endogenous Tip60 and ATF3 proteins could interact. We also determined whether ATF3 binds Tip60 under the DNA damage condition by carrying out pulldown assays, given that the ATF3 expression level varies largely before and after DNA-damage treatments [27] . We thus subjected HCT116-3 × FLAG cells to IR, and incubated cell lysates normalized to equal Tip60 or ATF3 level with GST–ATF3 or GST–Tip60 for pulldown assays [27] . The results show that ATF3 also interacted with Tip60 after DNA damage ( Fig. 1f , lanes 6–8, and Supplementary Fig. 1 , lanes 5 and 6). However, unlike the ATF3–p53 interaction [27] , the ATF3 binding to Tip60 did not appear to be altered by DNA damage induced by IR ( Fig. 1f and Supplementary Fig. 1 ). 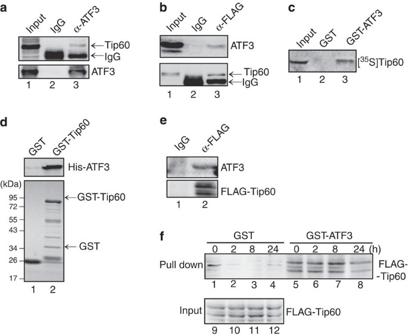Figure 1: ATF3 interacts with Tip60. (a,b) ATF3 interacted with Tip60 revealed by reciprocal co-IP assays. H1299 cells in 60-mm dishes were co-transfected with 3 μg of FLAG-Tip60 and 3 μg of ATF3, and subjected to co-IP using 1 μg of the ATF3 (a) or the FLAG antibody (b). (c) GST–ATF3 pulled downin vitro-translated Tip60. One microgram of GST–ATF3 or GST immobilized on 30 μl of glutathione agarose was incubated with 5 μl ofin vitro-translated [35S]-methionine-labelled Tip60 for GST-pulldown assays. (d) GST–Tip60 interacted with a purified ATF3 protein. Immobilized GST–Tip60 was incubated with 50 ng of recombinant ATF3 for GST pulldown assays. Upper, western blotting with the ATF3 antibody; lower, Ponceau S staining of the blot. (e) The interaction between the endogenous Tip60 and ATF3 proteins was confirmed by co-IP assays. HCT116 cells expressing a 3 × FLAG-tagged endogenous Tip60 protein were subjected to co-IP using the FLAG antibody. (f) Irradiation does not alter the binding of Tip60 to GST–ATF3. Lysates prepared from HCT116-3 × FLAG cells treated with 10 Gy of IR were incubated with 1 μg of immobilized GST–ATF3 or GST as indicated for pulldown assays. Tip60 was detected with the FLAG antibody. Figure 1: ATF3 interacts with Tip60. ( a , b ) ATF3 interacted with Tip60 revealed by reciprocal co-IP assays. H1299 cells in 60-mm dishes were co-transfected with 3 μg of FLAG-Tip60 and 3 μg of ATF3, and subjected to co-IP using 1 μg of the ATF3 ( a ) or the FLAG antibody ( b ). ( c ) GST–ATF3 pulled down in vitro -translated Tip60. One microgram of GST–ATF3 or GST immobilized on 30 μl of glutathione agarose was incubated with 5 μl of in vitro -translated [ 35 S]-methionine-labelled Tip60 for GST-pulldown assays. ( d ) GST–Tip60 interacted with a purified ATF3 protein. Immobilized GST–Tip60 was incubated with 50 ng of recombinant ATF3 for GST pulldown assays. Upper, western blotting with the ATF3 antibody; lower, Ponceau S staining of the blot. ( e ) The interaction between the endogenous Tip60 and ATF3 proteins was confirmed by co-IP assays. HCT116 cells expressing a 3 × FLAG-tagged endogenous Tip60 protein were subjected to co-IP using the FLAG antibody. ( f ) Irradiation does not alter the binding of Tip60 to GST–ATF3. Lysates prepared from HCT116-3 × FLAG cells treated with 10 Gy of IR were incubated with 1 μg of immobilized GST–ATF3 or GST as indicated for pulldown assays. Tip60 was detected with the FLAG antibody. Full size image ATF3 increases the Tip60 HAT activity As protein–protein interactions may alter the Tip60 HAT activity, we purified GST–Tip60 and carried out HAT activity assays using histone H4 and [ 3 H]-acetyl CoA. Whereas GST–Tip60 catalysed the transfer of the [ 3 H]-acetyl group to H4 as expected, recombinant ATF3 significantly increased the amount of acetylated H4 ( Fig. 2a ), indicating that ATF3 promoted the Tip60 HAT activity. Moreover, ATF3 appeared to increase the amount of [ 3 H]-acetylated Tip60 in a dose-dependent manner ( Fig. 2b , lanes 3–5 versus lane 2), suggesting that ATF3 also promoted Tip60 autoacetylation required for its HAT activity [12] , [29] . 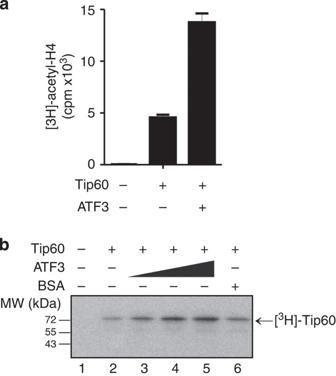Figure 2: ATF3 increases the Tip60 HAT activity. (a) ATF3 increased the Tip60 HAT activity. The Tip60 HAT activity was determined by incubating 0.5 μg of GST–Tip60 with 5 μl of [3H]-acetyl CoA, 0.5 μg of histone H4 and/or 1 μg of recombinant ATF3. The data are presented as mean±s.e.m. (n=3). (b) ATF3 promoted Tip60 autoacetylation. GST–Tip60 (0.5 μg) was incubated with H4, [3H]-acetyl CoA, ATF3 (0.5, 0.75 and 1 μg) or BSA (1 μg) as indicated, and subjected to SDS–PAGE followed by autography. Figure 2: ATF3 increases the Tip60 HAT activity. ( a ) ATF3 increased the Tip60 HAT activity. The Tip60 HAT activity was determined by incubating 0.5 μg of GST–Tip60 with 5 μl of [ 3 H]-acetyl CoA, 0.5 μg of histone H4 and/or 1 μg of recombinant ATF3. The data are presented as mean±s.e.m. ( n =3). ( b ) ATF3 promoted Tip60 autoacetylation. GST–Tip60 (0.5 μg) was incubated with H4, [ 3 H]-acetyl CoA, ATF3 (0.5, 0.75 and 1 μg) or BSA (1 μg) as indicated, and subjected to SDS–PAGE followed by autography. Full size image ATF3 increases Tip60 stability by blocking ubiquitination Tip60 is a relatively unstable protein and its stability can be altered by binding partners [12] . We thus tested whether ATF3 stabilizes Tip60. Co-expression of ATF3 increased the Tip60 expression level ( Fig. 3a , lane 2 versus lane 1). Conversely, knockdown of ATF3 expression using ATF3-specific short hairpin RNA (shRNA; shATF3) [28] resulted in decreased Tip60 expression in U2OS ( Fig. 3b ) and HCT116 cells ( Supplementary Fig. 2a ). These effects were unlikely caused by repression of Tip60 transcription as the Tip60 mRNA level was not decreased by shATF3 ( Fig. 3c and Supplementary Fig. 2b ). Rather, ATF3 increased the half-life of both the exogenously expressed ( Supplementary Fig. 2c ), and the endogenous Tip60 protein ( Fig. 3d and Supplementary Fig. 2d ). Together, these results argue for that ATF3 can stabilize Tip60. As the Tip60 stability is controlled by ubiquitin-mediated proteolysis [13] , [14] , we examined the Tip60 ubiquitination level in the absence or presence of ATF3. We found that ATF3 expression dramatically decreased the amount of ubiquitinated Tip60 protein ( Fig. 3e , lane 3 versus lane 2). Thus, ATF3 appeared to stabilize Tip60 by decreasing its ubiquitination level. 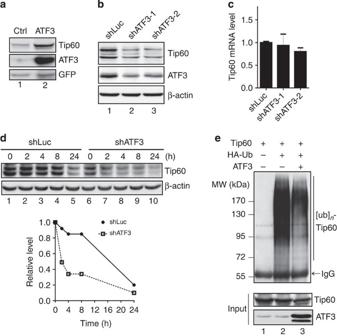Figure 3: ATF3 increases the Tip60 stability by decreasing its ubiquitination level. (a) ATF3 co-expression increased the Tip60 expression level. H1299 cells were transfected with 0.4 μg of FLAG-Tip60, 0.05 μg of GFP and/or 1.6 μg of ATF3 for 2 days, and then subjected to western blotting as indicated. The GFP expression levels across the samples were used to normalize transfection efficiency. (b,c) Knockdown of ATF3 expression decreased the protein level but not the mRNA level of Tip60. Two U2OS clones stably expressing shATF3 (shATF3-1 and shATF3-2) or the control shRNA (shLuc) were lysed for western blotting (b) or quantitative RT–PCR (c). The data are presented as mean±s.d. (n=3). (d) ATF3 knockdown decreased the Tip60 stability. U2OS cells expressing shATF3 or shLuc were treated with 100 μg ml−1of cycloheximide (CHX) and lysed for western blotting as indicated. Relative Tip60 levels were quantitated by densitometry and presented in the lower plot. (e) ATF3 expression decreased the Tip60 ubiquitination level. Lysates from H1299 cells transfected with 1 μg of FLAG-Tip60, HA-ubiquitin and/or ATF3 were subjected to immunoprecipitation using the FLAG antibody followed by SDS–PAGE. Ubiquitinated proteins were detected by western blotting using the HA antibody. Figure 3: ATF3 increases the Tip60 stability by decreasing its ubiquitination level. ( a ) ATF3 co-expression increased the Tip60 expression level. H1299 cells were transfected with 0.4 μg of FLAG-Tip60, 0.05 μg of GFP and/or 1.6 μg of ATF3 for 2 days, and then subjected to western blotting as indicated. The GFP expression levels across the samples were used to normalize transfection efficiency. ( b , c ) Knockdown of ATF3 expression decreased the protein level but not the mRNA level of Tip60. Two U2OS clones stably expressing shATF3 (shATF3-1 and shATF3-2) or the control shRNA (shLuc) were lysed for western blotting ( b ) or quantitative RT–PCR ( c ). The data are presented as mean±s.d. ( n =3). ( d ) ATF3 knockdown decreased the Tip60 stability. U2OS cells expressing shATF3 or shLuc were treated with 100 μg ml −1 of cycloheximide (CHX) and lysed for western blotting as indicated. Relative Tip60 levels were quantitated by densitometry and presented in the lower plot. ( e ) ATF3 expression decreased the Tip60 ubiquitination level. Lysates from H1299 cells transfected with 1 μg of FLAG-Tip60, HA-ubiquitin and/or ATF3 were subjected to immunoprecipitation using the FLAG antibody followed by SDS–PAGE. Ubiquitinated proteins were detected by western blotting using the HA antibody. Full size image ATF3 promotes USP7-mediated deubiquitination of Tip60 As it was recently shown that the deubiquitinase USP7 can remove polyubiquitin chains from Tip60 and stabilize the latter protein [17] , [30] , we tested whether ATF3 stabilizes Tip60 by promoting USP7 function. Whereas USP7 indeed increased the Tip60 expression level and concurrently decreased the amount of ubiquitinated Tip60, ATF3 expression promoted the effects of USP7 on Tip60 expression ( Fig. 4a , lanes 3 versus lane 2, and lane 5 versus lane 4) and ubiquitination ( Supplementary Fig. 3 , lane 3 versus lane 2), suggesting that ATF3 might promote USP7-mediated deubiquitination of Tip60. To directly test this possibility, we purified ubiquitinated Tip60 for in vitro deubiquitination assays to examine the catalytic activity of USP7 in the absence or presence of ATF3. As expected, recombinant USP7 catalysed removal of ubiquitin moieties from Tip60 ( Fig. 4b , lane 2 versus lane 1), and this effect was largely enhanced by ATF3 ( Fig. 4b , lane 3). As ATF3 alone did not appear to decrease the Tip60 ubiquitination level ( Fig. 4c , lane 3), these results argue for the notion that ATF3 promoted USP7-mediated deubiquitination of Tip60, thereby stabilizing the latter protein. To confirm that ATF3-mediated Tip60 stabilization was indeed through regulating USP7 activity, we treated the cells with a specific small-molecule USP7 inhibitor P5091 (ref. 31 ), and found that the ATF3 effects on Tip60 expression was significantly compromised in the cells where the USP7 activity was inhibited ( Fig. 4d , lane 4 versus lane 2). Similarly, inhibition of USP7 activity by P5091 (as evidenced by increased p53 expression [31] ), or knockdown of USP7 expression by short interfering RNA (siRNA), almost completely abolished shATF3-mediated downregulation of Tip60 expression ( Fig. 4e,f , lane 4 versus lane 3). Taken together, these results argue for that ATF3 likely stabilized Tip60 through promoting USP7-mediated deubiquitination of Tip60. 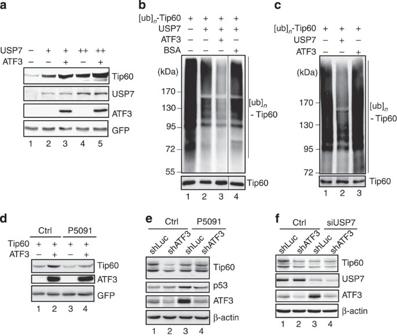Figure 4: ATF3 promotes USP7-mediated deubiquitination and stabilization of Tip60. (a) ATF3 promoted USP7-induced increase in Tip60 expression. H1299 cells were transfected with 0.4 μg of Tip60, 1.6 μg of ATF3, 0.05 μg of GFP and increasing amounts of USP7 (+, 0.4 μg; ++, 0.8 μg) as indicated, and then lysed for western blotting. (b) ATF3 promoted USP7-mediated deubiquitination of Tip60. Ubiquitinated Tip60 was purified by the FLAG affinity chromatography from 293T cell lysates transfected with FLAG-Tip60 and HA-ubiquitin. The ubiquitinated protein was pre-incubated with 1 μg of ATF3 or BSA on ice, and then mixed with 1 μg of USP7 forin vitrodeubiquitination assays. Tip60 ubiquitination was determined by the HA antibody. (c) ATF3 did not directly deubiquitinate Tip60. Ubiquitinated Tip60 was incubated with ATF3 or USP7 forin vitrodeubiqutination assays. (d) P5091 diminished ATF3-induced increase in Tip60 expression. H1299 cells transfected with 0.4 μg of Tip60 and/or 1.6 μg of ATF3 were treated with or without 30 μM of P5091 overnight, and then subjected to western blotting. (e) P5091 abolished the decrease in Tip60 expression caused by shATF3. U2OS cells expressing shLuc or shATF3 were treated with 30 μM of P5091, and then lysed for western blotting using indicated antibodies. (f) USP7 inhibition by siRNA abolished shATF3-medidated downregulation of Tip60 expression. shATF3- or shLuc-U2OS cells were transfected with 100 pmol of siUSP7 for 3 days and then lysed for western blotting. Figure 4: ATF3 promotes USP7-mediated deubiquitination and stabilization of Tip60. ( a ) ATF3 promoted USP7-induced increase in Tip60 expression. H1299 cells were transfected with 0.4 μg of Tip60, 1.6 μg of ATF3, 0.05 μg of GFP and increasing amounts of USP7 (+, 0.4 μg; ++, 0.8 μg) as indicated, and then lysed for western blotting. ( b ) ATF3 promoted USP7-mediated deubiquitination of Tip60. Ubiquitinated Tip60 was purified by the FLAG affinity chromatography from 293T cell lysates transfected with FLAG-Tip60 and HA-ubiquitin. The ubiquitinated protein was pre-incubated with 1 μg of ATF3 or BSA on ice, and then mixed with 1 μg of USP7 for in vitro deubiquitination assays. Tip60 ubiquitination was determined by the HA antibody. ( c ) ATF3 did not directly deubiquitinate Tip60. Ubiquitinated Tip60 was incubated with ATF3 or USP7 for in vitro deubiqutination assays. ( d ) P5091 diminished ATF3-induced increase in Tip60 expression. H1299 cells transfected with 0.4 μg of Tip60 and/or 1.6 μg of ATF3 were treated with or without 30 μM of P5091 overnight, and then subjected to western blotting. ( e ) P5091 abolished the decrease in Tip60 expression caused by shATF3. U2OS cells expressing shLuc or shATF3 were treated with 30 μM of P5091, and then lysed for western blotting using indicated antibodies. ( f ) USP7 inhibition by siRNA abolished shATF3-medidated downregulation of Tip60 expression. shATF3- or shLuc-U2OS cells were transfected with 100 pmol of siUSP7 for 3 days and then lysed for western blotting. Full size image The ATF3–Tip60 interaction is required for regulating Tip60 We next addressed the question as to whether the ATF3-mediated regulation of Tip60 was due to its interaction with Tip60. Towards this end, we first defined the domains required for the ATF3–Tip60 interaction using GST-pulldown assays. The results indicate that ATF3 bound Tip60 at a region adjacent to the HAT domain (aa 111–212) as neither the Tip60 N-terminal fragment (aa 1–110) nor the C-terminal HAT-containing fragment (aa 213–513) could pull down ATF3 ( Fig. 5a and Supplementary Fig. 5 ). On the other hand, Tip60 bound ATF3 at its C-terminal region (aa 81–181) that contains the characteristic basic-region leucine zipper domain domain ( Fig. 5b , lane 5). Moreover, deletion of the leucine zipper (Zip) subdomain (Δ102–139, or ΔATF3) almost completely abolished the ATF3–Tip60 binding ( Fig. 5b , lane 6 and Supplementary Fig. 4 , lane 4), indicating that the ATF3 Zip domain required for interacting with many other proteins [22] , [23] , [27] also mediated the Tip60–ATF3 interaction. We therefore tested whether this Tip60-binding-deficient protein loses the ability to regulate Tip60. Indeed, recombinant ΔATF3 failed to increase the Tip60 acetyltransferase activity as evidenced by the lack of increase in the Tip60 autoacetylation level ( Fig. 5c , lane 4 versus lane 3). Similarly, the mutant protein failed to increase the expression level ( Fig. 5d , lane 3 versus lane 2) or decrease the ubiquitination level of Tip60 ( Fig. 5e , lane 3 versus lane 2). Moreover, in vitro deubiquitination assays revealed that ΔATF3 lost the activity to promote USP7-mediated deubiquitination of Tip60 ( Fig. 5f , lane 4 versus lane 3). These results argue for the notion that the ATF3 binding to Tip60 increases its HAT activity and stabilizes the HAT. 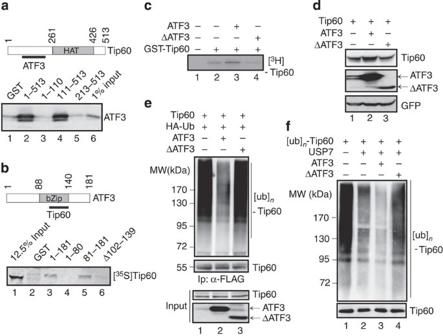Figure 5: The ATF3–Tip60 interaction is required for Tip60 regulation. (a) GST-pulldown assays defined Tip60 regions for ATF3 binding. One microgram of indicated Tip60-truncated proteins fused to GST were immobilized on glutathione agarose and incubated with 5 μl ofin vitro-translated ATF3 for GST-pulldown assays. The pulldown proteins were detected by western blotting using the ATF3 antibody. Ponceau S staining of the blot is shown inSupplementary Fig. 5. (b) GST-pulldown assays defined ATF3 regions required for Tip60 binding. Indicated ATF3 fragments (1 μg) were fused with GST, and were incubated with [35S]-labelled Tip60 for GST-pulldown assays. (c) The Tip60-binding-deficient mutant (ΔATF3) lost the activity to promote Tip60 autoacetylation. The experiments were carried out as described inFig. 2b. (d) ΔATF3 failed to increase the Tip60 expression level. H1299 cells were transfected with 0.4 μg of Tip60, and 1.6 ATF3 or ΔATF3 as indicated for western blotting. (e) ΔATF3 did not decrease the Tip60 ubiquitination level as shown by western blotting. The experiments were carried out as described inFig. 3e. (f) Recombinant ΔATF3 failed to promote USP7-mediated deubiquitination of Tip60 as determined byin vitrodeubiquitination assays as inFig. 4b. Figure 5: The ATF3–Tip60 interaction is required for Tip60 regulation. ( a ) GST-pulldown assays defined Tip60 regions for ATF3 binding. One microgram of indicated Tip60-truncated proteins fused to GST were immobilized on glutathione agarose and incubated with 5 μl of in vitro -translated ATF3 for GST-pulldown assays. The pulldown proteins were detected by western blotting using the ATF3 antibody. Ponceau S staining of the blot is shown in Supplementary Fig. 5 . ( b ) GST-pulldown assays defined ATF3 regions required for Tip60 binding. Indicated ATF3 fragments (1 μg) were fused with GST, and were incubated with [ 35 S]-labelled Tip60 for GST-pulldown assays. ( c ) The Tip60-binding-deficient mutant (ΔATF3) lost the activity to promote Tip60 autoacetylation. The experiments were carried out as described in Fig. 2b . ( d ) ΔATF3 failed to increase the Tip60 expression level. H1299 cells were transfected with 0.4 μg of Tip60, and 1.6 ATF3 or ΔATF3 as indicated for western blotting. ( e ) ΔATF3 did not decrease the Tip60 ubiquitination level as shown by western blotting. The experiments were carried out as described in Fig. 3e . ( f ) Recombinant ΔATF3 failed to promote USP7-mediated deubiquitination of Tip60 as determined by in vitro deubiquitination assays as in Fig. 4b . Full size image ATF3 knockdown impairs ATM activation by DNA damage As Tip60 can sense DNA double-strand breaks and acetylate ATM for its autophosphorylation and subsequent activation [3] , we immunoprecipitated ATM from ATF3 knockdown cells and determined its acetylation level using an acetyl-lysine antibody. Whereas IR indeed induced ATM acetylation ( Fig. 6a , lane 2 versus lane 1), the amount of acetylated ATM protein was dramatically decreased in the shATF3-expressing cells ( Fig. 6a , lane 4 versus lane 2). Consistent with these results, IR-induced phosphorylation of ATM at serine 1981 was dramatically suppressed in the ATF3 knockdown U2OS cells where the Tip60 expression level was downregulated ( Fig. 6b , lanes 9–14 versus lanes 2–7). Similarly, IR-induced phosphorylation of ATM substrates including H2AX, Chk2 and p53 was also inhibited in the shATF3 cells ( Fig. 6b ). The suppression of ATM activation by shATF3 was not limited to U2OS cells, nor was it due to clonal variation or off-target effects of shRNA, as we also found impaired ATM signalling in ATF3 downregulated HCT116 cells ( Fig. 6c ), another shATF3-expressing U2OS clone ( Supplementary Fig. 6 ), and HCT116 cells engineered to lose ATF3 expression by homologous recombination ( Supplementary Fig. 7a ). Moreover, ATM activation in response to a sublethal dose of IR (2 Gy) was also impaired in ATF3 knockdown U2OS cells ( Supplementary Fig. 8a ). These results thus indicate that ATF3 is required for ATM activation in response to IR. The observations that the total p53 level was downregulated in the shATF3 cells ( Fig. 6b,c and Supplementary Fig. 8a ) are in line with our early finding that ATF3 can stabilize p53 (ref. 27 ). Although IR dramatically induced ATF3 expression in the control (shLuc) cells, it is important to note that neither the Tip60 expression level ( Fig. 6b,c ) nor the Tip60 ubiquitination level ( Supplementary Fig. 9a ) was significantly altered by IR. These seemingly inconsistent results could be explained by the findings that ATF3-mediated Tip60 stabilization was USP7-dependent ( Fig. 4 ) and that USP7 expression was decreased by IR ( Supplementary Fig. 9b ) as previously reported [32] . 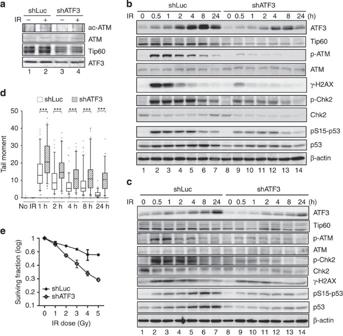Figure 6: Knockdown of ATF3 expression leads to impaired ATM activation by IR. (a) IR-induced ATM acetylation was diminished by ATF3 knockdown. U2OS cells expressing shLuC or shATF3 were subjected to 10 Gy of γ-irradiation. ATM was then immunoprecipitated using an ATM antibody, and its acetylation level was determined by western blotting using the acetyl-lysine antibody. (b,c) IR-induced activation of ATM and phosphorylation or ATM substrates were impaired in ATF3 knockdown U2OS (b) and HCT116 cells (c). Cells expressing shLuc or shATF3 were irradiated (10 Gy), and then subjected to western blotting using the indicated antibodies. (d) Neutral comet assays show accumulation of DNA lesions in shATF3-expressing U2OS cells. Cells were irradiated by 10 Gy of γ-rays and used for comet assays after indicated time. ***P<0.001, Mann–WhitneyU-test. (e) ATF3 knockdown sensitized U2OS cells to IR-induced cell death. Irradiated cells were plated in 100-mm dishes in triplicate and subjected to colony formation assays. Figure 6: Knockdown of ATF3 expression leads to impaired ATM activation by IR. ( a ) IR-induced ATM acetylation was diminished by ATF3 knockdown. U2OS cells expressing shLuC or shATF3 were subjected to 10 Gy of γ-irradiation. ATM was then immunoprecipitated using an ATM antibody, and its acetylation level was determined by western blotting using the acetyl-lysine antibody. ( b , c ) IR-induced activation of ATM and phosphorylation or ATM substrates were impaired in ATF3 knockdown U2OS ( b ) and HCT116 cells ( c ). Cells expressing shLuc or shATF3 were irradiated (10 Gy), and then subjected to western blotting using the indicated antibodies. ( d ) Neutral comet assays show accumulation of DNA lesions in shATF3-expressing U2OS cells. Cells were irradiated by 10 Gy of γ-rays and used for comet assays after indicated time. *** P <0.001, Mann–Whitney U -test. ( e ) ATF3 knockdown sensitized U2OS cells to IR-induced cell death. Irradiated cells were plated in 100-mm dishes in triplicate and subjected to colony formation assays. Full size image Defective ATM activation would result in impaired cellular response to IR-induced DNA damage. Indeed, we found that more DNA lesions were accumulated in the shATF3 cells than in the shLuc cells ( Fig. 6d and Supplementary Fig. 8b ), or accumulated in ATF3 knockout cells than in the wild-type HCT116 cells ( Supplementary Fig. 7b ). Moreover, knockdown of ATF3 expression sensitized cells to IR-induced death ( Fig. 6e ). Our results thus suggest that ATF3 promoted ATM activation and this effect was likely through sustaining Tip60 activity. ATF3 promotes ATM signalling in a Tip60-dependent manner To test whether the promotion of ATM activation by ATF3 was through regulating Tip60, we knocked down Tip60 expression by siRNA and determined IR-induced ATM activation. Consistent with the pivotal role of Tip60 in ATM activation [3] , [4] , even a modest downregulation of Tip60 expression was sufficient to suppress IR-induced phosphorylation of ATM and H2AX in the control cells ( Fig. 7a , lane 4 versus lane 2). However, the extents of shATF3-mediated suppression of ATM activation (that is, shATF3-mediated downregulation of p-ATM and γ-H2AX levels) were decreased in the cells where Tip60 expression was knocked down ( Fig. 7a , comparing lane 6 and lane 2 with lane 8 and lane 4). Similarly, whereas Tip60 knockdown led to accumulation of DNA lesions and radiosensitivity as expected, shATF3 appeared to be less effective in accumulating damaged DNA or increasing sensitivity to IR-induced death in the siTip60-knockdown cells ( Fig. 7b,c ). These results suggest that shATF3-mediated suppression of ATM signalling was likely to be dependent on Tip60. Therefore, in addition to directly activating p53 (ref. 27 ), ATF3 appears to regulate Tip60 activity and promote subsequent ATM signalling required for the maintenance of genomic stability on genotoxic insults ( Fig. 7d ). 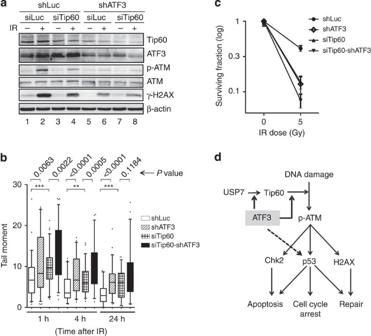Figure 7: ATF3 promotes ATM signalling through regulating Tip60. (a) shATF3-mediated suppression of ATM activation was compromised in cells expressing Tip60 siRNA. shLuc- or shATF3-expressing U2OS cells were transfected with 100 pmol of Tip60 siRNA (siTip60) or control siRNA (siLuc) for 3 days, and then subjected to 10 Gy of γ-irradiation for western blotting using the indicated antibodies. (b,c) shATF3 had less effect on inducing DNA lesion accumulation and radiosensitivity in siTip60-expressing cells. Irradiated U2OS cells were subjected to neutral comet assays (b) or colony formation assays (c) as described inFig. 6d,e. **P<0.01; ***P<0.001;P-values were calculated by Mann–WhitneyU-test. (d) Schematic diagram showing the model whereby ATF3 regulates the HAT activity of Tip60 while promoting USP7-mediated deubiquitination of Tip60, and thereby activates ATM signalling on DNA damage. Figure 7: ATF3 promotes ATM signalling through regulating Tip60. ( a ) shATF3-mediated suppression of ATM activation was compromised in cells expressing Tip60 siRNA. shLuc- or shATF3-expressing U2OS cells were transfected with 100 pmol of Tip60 siRNA (siTip60) or control siRNA (siLuc) for 3 days, and then subjected to 10 Gy of γ-irradiation for western blotting using the indicated antibodies. ( b , c ) shATF3 had less effect on inducing DNA lesion accumulation and radiosensitivity in siTip60-expressing cells. Irradiated U2OS cells were subjected to neutral comet assays ( b ) or colony formation assays ( c ) as described in Fig. 6d,e . ** P <0.01; *** P <0.001; P -values were calculated by Mann–Whitney U -test. ( d ) Schematic diagram showing the model whereby ATF3 regulates the HAT activity of Tip60 while promoting USP7-mediated deubiquitination of Tip60, and thereby activates ATM signalling on DNA damage. Full size image Emerging as a key regulator of the DNA damage response, Tip60 facilitates DNA repair and determines cell fate by acetylating histones, p53 and ATM, thereby activating signalling required for mounting appropriate cellular response to DNA damage [1] , [3] , [7] , [8] . Whereas many of the Tip60-regulated events have been elucidated, little is known about how the Tip60 activity is regulated. Here we identified ATF3 as one of the few Tip60 regulators that can interact with Tip60 and increase both the HAT activity and the stability of the major ATM activator. Thus, IR-induced ATM acetylation and activation were suppressed leading to impaired DNA damage response in cells where the ATF3 function was compromised ( Fig. 6 ). Given that DNA damage conferred by various stimuli can generally induce ATF3 expression, our study has therefore revealed a common mechanism by which the cell may utilize to maintain genomic integrity in the face of intrinsic and/or environmental genotoxic insults ( Fig. 7e ). This common mechanism appeared to be independent of the transcription activity of ATF3, but require the binding of ATF3 to Tip60—a reminiscence of our earlier findings that ATF3 activates p53 while repressing the androgen receptor through protein–protein interactions [23] , [27] . Our results are in line with the notion that the common stress-inducible transcription factor contributes to the DNA damage response through mechanisms apart from direct transcriptional regulation. A direct consequence of the ATF3–Tip60 interaction was the promotion of the Tip60 HAT activity. This effect is contrary to that of ATF2, an ATF3 relative that binds Tip60 at a region (aa 368–513) overlapping with the acetyl CoA-binding site, thereby inhibiting the Tip60 HAT activity [14] . ATF3 rather bound Tip60 at a region (aa 111–212) adjacent to the HAT domain, and was thus likely to alter the conformation of the HAT domain to a state in favour of the catalytic activity. Indeed, like p300 (ref. 33 , conformational changes of the HAT domain caused by post-translational modifications (for example, autoacetylation) were shown to prevent Tip60 from oligomerization, thereby increasing substrate-binding and the HAT activity [29] . Interestingly, ATF3 promoted not only acetylation of tested Tip60 substrates (for example, H4, ATM), but Tip60 autoacetylation ( Fig. 2b ). The latter effect might further alter the conformation of the HAT domain [12] , [29] , thereby increasing the Tip60 HAT activity to ensure maximal activation of Tip60 by ATF3. Acetylation of Tip60 at the HAT domain may also prevent ubiquitin-mediated protein degradation and thus increase the Tip60 stability [12] . However, the promotion of Tip60 autoacetylation by ATF3 is unlikely the only mechanism by which ATF3 stabilized Tip60. Rather, we found that ATF3 promoted USP7-mediated deubiquitination of Tip60, thereby diminishing Tip60 ubiquitination required for proteosomal degradation. Indeed, a USP7-specific inhibitor or USP7 siRNA could abolish the effects of ATF3 on Tip60 ( Fig. 4e,f ), arguing for the notion that ATF3-mediated Tip60 stabilization is dependent on USP7. USP7 is the only known deubiquitinase capable of removing ubiquitin chains from Tip60 (refs 17 , 30 ), whereas it can also regulate stabilities of other proteins involved in the DNA damage response (for example, MDM2 and p53) [19] . As ATF3 appears to bind to MDM2 as well as p53 (refs 27 , 28 ), the observation that ATF3 promoted USP7-mediated deubiquitination of Tip60 suggests a possibility that ATF3 might also regulate the MDM2 or p53 stability through regulating USP7 in the DNA damage response. However, it was unlikely that ATF3 directly regulates the USP7 deubiquitinase activity as pre-incubation of ATF3 with the ubiquitinated Tip60 protein, but not with USP7, appeared to be required for the ATF3 deubiquitination-promoting effect as revealed by the in vitro ubiquitination assays ( Supplementary Fig. 10A ). Likewise, ATF3 did not appear to promote Tip60 deubiquitination by facilitating USP7 substrate-binding since ATF3 expression did not enhance the USP7–Tip60 interaction ( Supplementary Fig. 10b ). Our results rather suggest that the Tip60 conformational change induced by ATF3 binding might expose the ubiquitin chains for ready access to USP7, thereby promoting the removal of the ubiquitin moieties from Tip60. Interestingly, both the USP7 inhibitor and the USP7 siRNA appeared to increase ATF3 expression ( Fig. 4e,f , lane 3). While USP7 inhibition could result in downregulation of MDM2 (ref. 19 ), thereby preventing ATF3 from MDM2-mediated ubiquitination and degradation [28] , it might also be that the increased ATF3 expression was caused by USP7-catalysed deubiquitination of ATF3. While this intriguing possibility awaits a test, these results suggest that USP7 might contribute to ATF3 induction and play a previously unidentified role in the DNA damage response. A major mechanism by which Tip60 regulates the DNA damage response is to activate ATM, which in turn directly or indirectly phosphorylates p53 at multiple sites including serine 15 and serine 20, thereby activating p53 to promote cell cycle arrest or induce apoptosis. In addition, Tip60 can directly acetylate p53 at lysine 120 (K120) and promote transactivation of pro-apoptotic genes (for example, Bax, PUMA) [7] , [8] . Consistent with the role of ATF3 in regulating Tip60, knockdown of ATF3 expression resulted in decreased p53 phosphorylation ( Fig. 6b,c ). As ATF3 could increase the HAT activity of Tip60 ( Fig. 2 ), one would expect that ATF3 might promote p53 K120 acetylation in response to DNA damage. To our surprise, we found that ATF3 deficiency did not suppressed but rather modestly enhanced p53 K120 acetylation induced by etoposide ( Supplementary Fig. 11a , lanes 4–6 versus lanes 1–3). Further experiments revealed that ATF3 partially prevented Tip60 from binding to p53 ( Supplementary Figs 11b and 12c ), which might explain why elevated p53 K120 acetylation was detected in ATF3-deficient cells. However, we found that ATF3 was still capable of promoting p53 transcriptional activity leading to increased expression of p21 and PUMA in the tested cells ( Supplementary Fig. 11d ). Therefore, ATF3 appears to activate p53 through two distinct mechanisms, that is, stabilizing p53 by blocking its ubiquitination [27] , and promoting Tip60 function and subsequent activation of ATM signalling ( Fig. 7e ). Cell culture and colony formation assays U2OS, HCT116 and H1299 cells were originally from ATCC, and cultured in DMEM, McCoy’s 5A and RPMI 1640 medium supplemented with 10% fetal bovine serum, respectively. HCT116-3 × Flag-Tip60 cells were obtained from Dr. Zhenghe Wang [18] and cultured in McCoy’s 5A medium. Transfections were carried out using Lipofectamine 2000 (Invitrogen) according to the manufacturer’s instruction. For colony formation assays, 200 cells plated in six-well plates were irradiated by IR, and surviving colonies were fixed with 10% formalin and stained with 0.1% of crystal violet 10 days later. GST-pulldown and co-IP assays For GST-pulldown assays, 1 μg of GST or GST fusion proteins immobilized on glutathione agarose (Sigma) were incubated with in vitro -translated proteins (5 μl) or recombinant proteins (50 ng) in a buffer containing 20 mM Tris-HCl, pH 8.0, 100 mM NaCl, 2 mM EDTA, 2 mM dithiothreitol (DTT), 5% glycerol and 0.4% NP-40 at 4 °C overnight, followed by extensive washes with a similar buffer containing 150 mM NaCl. Bound proteins were eluted by boiling in the loading buffer and detected by western blotting or fluorography. For co-IP assay, cell lysates (1–2 mg) were incubated with 1 μg of the ATF3 antibody or FLAG antibody in RIPA buffer (50 mM Tris-HCl, pH 7.4, 100 mM NaCl, 1% NP-40, 0.1% SDS, 0.5% sodium deoxycholate and 1 mM EDTA) at 4 °C overnight. Protein A or protein G agarose (30 μl; Roche) were then added and incubated at 4 °C for 5 h. After extensive washes with RIPA buffer containing 150 mM NaCl, precipitated proteins were eluted and detected using western blotting. The p-Ser1981 ATM (no. 5883, 1:1,000), γ-H2AX (no. 2557, 1:1,000), α-Chk2 (no. 2197, 1:1,000), Chk2 (no. 6334, 1:1,000) and p-Ser15 p53 (no. 9284, 1:1,000), acetylated-lysine antibody (no. 9441, 1:1,000) were purchased from Cell Signaling. The HA (sc-7392, 1:200), the ATF3 (sc-188, 1: 1,000), and the p53 DO-1 (sc-126, 1:1,000) antibodies were from Santa Cruz, whereas the USP7 (NB110-513, 1:10,000), FLAG (F3165, 1:4,000) and ATM (Ab-3, 2 μg ml −1 ) antibodies were from Novus, Sigma and Millipore, respectively. The Tip60 antibody (1:1,000) was a kind gift from Dr. Bruno Amati [9] . Uncropped images of western blots are shown in Supplementary Fig. 12 . HAT activity assays GST–Tip60 was purified by glutathione agarose beads using a standard protocol [7] . Custom purification of His-ATF3 or His-ΔATF3 through a two-step protocol (IMAC affinity chromatography followed by SEC FPLC) was carried out by ProteinOne. The Tip60 HAT activity was assayed by incubating 0.5 μg of GST–Tip60 with 5 μl of [ 3 H]-acetyl CoA (PerkinElmer) and 0.5 μg of recombinant histone H4 (Biolabs) with or without purified ATF3 in a buffer containing 50 mM Tri-HCl (pH 8.0), 1 mM DTT, 0.1 mM EDTA and 10% glycerol for 1 h at 30 °C. Reaction mixtures were spotted on P81 cellulose papers (Millipore) and the papers were washed for six times with 50 ml of 50 mM sodium phosphate (pH 9.0). After the final wash, the cellulose papers were air-dried and radioactivity was measured using a scintillation counter (Beckman). To measure Tip60 autoacetylation, reaction mixtures were resolved using SDS–PAGE, and the [ 3 H]-acetyl-labelled Tip60 was visualized using autography. Ubiquitination assays and in vitro deubiquitination assays For ubiquitination assays, H1299 cells transfected with FLAG-Tip60 and HA-ubiquitin with or without ATF3 or USP7 were treated with 5 μM of MG132 overnight, and then lysed in the FLAG lysis buffer (50 mM Tris-HCl, pH 7.9, 137 mM NaCl, 10 mM NaF, 1 mM EDTA, 1% Triton X-100, 0.2% sarkosyl and 10% glycerol). Cell lysates (1–2 mg) were incubated with 20 μl of anti-FLAG M2 affinity gel (Sigma) at 4 °C overnight. After extensive washes, agarose gels were loaded on spin columns (Affymetrix), and bound FLAG-Tip60 was eluted with 20 μl of FLAG peptide at a final concentration of 0.1 mg ml −1 . Tip60 ubiquitination was determined by western blotting using the haemagglutinin (HA) antibody [27] , [28] . For deubiquitination assays, ubiquitinated Tip60 was first purified from 293T cells transfected with FLAG-Tip60 and HA-ubiquitin using the anti-FLAG M2 affinity gel as described above. After pre-incubated with 1 μg of ATF3, ΔATF3 or bovine serum albumin (BSA), on ice for 2 h, ubiquitinated Tip60 (1 μl) was mixed with 0.75 μg of His-USP7 (Boston Biochem) and incubated in a buffer containing 50 mM Tris-HCl, pH 8.0, 50 mM NaCl, 1 mM EDTA, 5% glycerol and 10 mM fresh DTT at 37 °C for 3 h (ref. 17 ). The reactions were then subjected to western blotting for detection of ubiquitination using the HA antibody. siRNA/shRNA knockdown and quantitative PCR Knockdown of ATF3 expression was carried out using the pSIH-H1 shRNA Cloning and Lentivector Expression system (System Biosciences) following the manufacturer’s protocol. The ATF3-targeted sequence was 5′- GCAAAGTGCCGAAACAAGA -3′ and 5′- GAGAAACCTCTTTATCCAA -3′ as previously described [22] . The Tip60 siRNA was synthesized on the basis of an earlier publication [7] , and the targeted sequence was 5′- ACGGAAGGTGGAGGTGGTT -3′. For reverse transcriptase (RT)–PCR, total RNA was extracted from cells using Trizol (Invitrogen), and then reverse-transcribed for real-time PCR assays using the SYBR Green reagents [34] . The Tip60 primer sequences are 5′- GGGGAGATAATCGAGGGCTG -3′ and 5′- TCCAGACGTTTGTTGAAGTCAAT -3′. Neutral comet assay Irradiated cells were trypsinized, centrifuged for 2 min at 300 g and resuspended in PBS at 2 × 10 4 ml −1 . Cell suspensions were then mixed with 1% of low-melting-point agarose at 1:3 (V/V) and layered on a microscope slide pre-coated with 1% of agarose gel. Cells in gels were lysed with the neutral lysis buffer (2 M NaCl, 30 mM EDTA, 10 mM Tris-HCl, pH 8.5, 1% N-laurylsarcosine and 1% Triton X-100) at 4 °C for 1 h. After three times of rinses with the TBE buffer (90 mM Tris, 90 mM boric acid and 2 mM EDTA, pH 8.5) at room temperature for 30 min, slides were submerged in TBE for electrophoresis at 20 V for 25 min. Slides were then rinsed, neutralized in distilled water, dipped in ethanol and dried. Slides were stained using 2.5 μg ml −1 of ethidium bromide in distilled water for 20 min and observed under a fluorescence microscope. At least 100 comet images from each slide were analysed using the CASP software ( http://casplab.com/ ). How to cite this article: Cui, H. et al . The stress-responsive gene ATF3 regulates the histone acetyltransferase Tip60. Nat. Commun. 6:6752 doi: 10.1038/ncomms7752 (2015).